Reply to: Revisiting the identification ofSyllipsimopodi bideniand timing of the decabrachian-octobrachian divergence 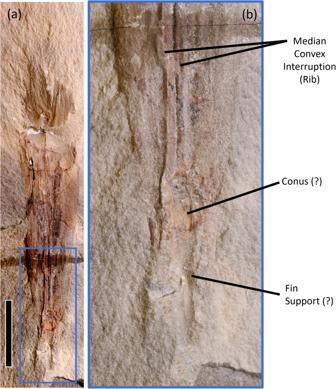Fig. 1:Syllipsimopodi bideniholotype ROMIP 64897. aFull specimen; scale = 1 cm.bBoxed region of Fig. 1a, showing posterior/apex. Note the pronounced median convex interruption (posteriorly bipartite rib), possible conus, and possible fin support; also note the absence of septa and a primordial rostrum (compare to Fig.2c). Color differences between images caused by lighting angle. 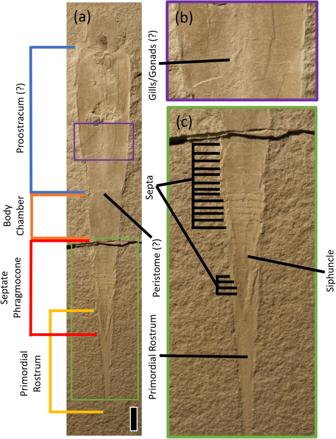Fig. 2:Gordoniconus beargulchensisholotype AMNH 43264, part. aComplete specimen, showing suggested proostracum (blue), body chamber (orange), septate phragmocone (red) and primordial rostrum (yellow); scale = 1 cm.bPurple boxed region of Fig.1a, showing structure interpreted as gills/gonads.cGreen boxed posterior region of Fig.1a, showing phragmocone and primordial rostrum; note the thin siphuncle and numerous complete septa, not all are marked. Image credit: S. Thurston. The holotypes, ROMIP 64897 and AMNH 43264/50267, were observed using a hand lens and under a light microscope at the American Museum of Natural History. The photograph for Fig. 1a was taken using a Canon EOS 60D camera with an EF-S60mm f/2.8 Macro USM lens and a Hoya 52 mm Circular Polarizing Pro 1 digital multi-coated glass filter; Cognisys Stackshot 3X Macro Rail Package and Helicon Focus 6.7.1 Pro were used to z-stack images. Photographs for Fig. 1b and Fig. 2 were taken using a Nikon D300 camera. Composite images were stitched using Adobe Photoshop 2021. All measurements were taken using ImageJ.